An artificial primitive mimic of the Gramicidin-A channel Gramicidin A (gA) is the simplest known natural channel, and important progress in improving conduction activity has previously been obtained with modified natural gAs. However, simple artificial systems mimicking the gA functions are unknown. Here we show that gA can be mimicked using a simple synthetic triazole or ‘T-channel’ forming compound (TCT), having similar constitutional functions as the natural gAs. As in gA channels, the carbonyl moieties of the TCT, which point toward the T-channel core and surround the transport direction, are solvated by water. The net-dipolar alignment of water molecules along the chiral pore surfaces influences the conduction of protons/ions, envisioned to diffuse along dipolar hydrophilic pathways. Theoretical simulations and experimental assays reveal that the conduction through the T-channel, similar to that in gA, presents proton/water conduction, cation/anion selectivity and large open channel-conductance states. T-channels—associating supramolecular chirality with dipolar water alignment—represent an artificial primitive mimic of gA. Transmembrane protein channels operate the collective information stored in sets of building constituents to achieve specific functional behaviours [1] , [2] , [3] , [4] , [5] , [6] , [7] , [8] , [9] . The constitutional topography of the pores provides hydrophilic pathways for translocation of electrolytes involved in vital cellular processes, including ion transport across epithelia to electrical signal production in neurons. The questions as to how the electrolytes diffuse along the protein channels and through the selectivity filters have been previously answered. Electrostatic considerations have been shown to play an important effect in the selectivity of Gramicidin A (gA) [1] , [2] , [3] , Aquaporin [4] , KCsAK + (ref. 5 ) and M2-Influenza A [6] , [7] , [8] channels. Among these non-exclusive examples of protein channels the best characterized one is gA in which ions, protons and water molecules are envisioned to diffuse along a single-file column filling the pore. Water, an electrically dipolar molecule, can influence, by its dynamic alignment, ionic/proton conduction, ion-valence selectivity and the other properties of the gA channel [1] , [2] , [3] . The ability to encapsulate water clusters in artificial systems might offer possibilities to explore water behaviours very close to pore-confined biological water and exhibiting properties at the limits between solid and liquid states. Despite the impressive development of entrapping water clusters by complex superstructures, only few artificial systems have been used to selectively transport water efficiently through bilayer membranes [10] , [11] , [12] , [13] , [14] . Understanding the molecular-scale hydrodynamics of water and ions confined within simple artificial systems has crucial relevance for many biological events. Here we show that a bola-amphiphile-triazole compound ( TCT ) undergoes self-assembly via multiple H-bonds to form stable pores in bilayers. Such self-assembled pores display diastereoisomeric chiral internal hypersurfaces on which oriented dipolar water-wire arrays can form. This system, which can be viewed as a primitive gA mimic, also presents ion/proton and water-channel conductance states in lipid bilayer membranes. Synthesis and self-assembly of TCT compound The 1,6-diisocyanatohexane, 1 , was treated with two equivalents of 3-amino-1,2,4-triazole, 2 , to afford TCT as a white powder ( Fig. 1 and Supplementary Fig.1 ). It is important to note that subsequent reactions under the same experimental setup, between non-stoichiometric mixtures of 1 and 2 (1:1, 1:2 or 1:3, mol:mol) always afforded pure compound TCT . A doubly substituted triazole-N-CONH and amino-NHCONH compound was never observed as side products, probably due to the very low reactivity of the amino guanidinium-type group of 2 . The 1 H, 13 C-NMR and electrospray ionization–mass spectrometry are in agreement with the unexpected reaction pathway. 1 H NMR dilution experiments conducted on CDCl 3 solutions showed practically insignificant downfield shift of NH protons on increasing concentration ( Supplementary Note 1 and Supplementary Fig. 2 ), which is indicative of a strong self-association of TCT through the intermolecular hydrogen bonding in solution. 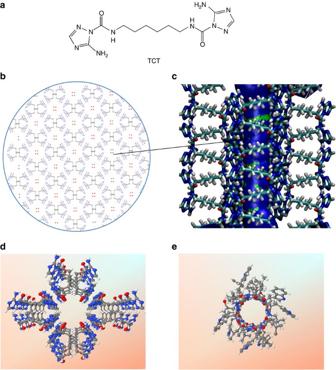Figure 1: Molecular structures and crystal packing. (a) Chemical formula ofTCT. (b) Top and (c) side views in line and stick representation, respectively, of the T-channels; the water molecules are shown as (b) red dots and (c) the Van der Waals surface of the pore is shown as a blue surface. The latter was calculated by the HOLE programme, which was first applied to the Gramicidin pore9. Pore structures of (d) T-channel and (e) Gramicidine A (gA) at the same dimensional scale. The gA coordinates were taken from the literature2. Red ellipsoids (forTCT) or balls (for gA) designate oxygen atoms, blue for nitrogen, grey for carbon and white for hydrogen. Figure 1: Molecular structures and crystal packing. ( a ) Chemical formula of TCT . ( b ) Top and ( c ) side views in line and stick representation, respectively, of the T-channels; the water molecules are shown as ( b ) red dots and ( c ) the Van der Waals surface of the pore is shown as a blue surface. The latter was calculated by the HOLE programme, which was first applied to the Gramicidin pore [9] . Pore structures of ( d ) T-channel and ( e ) Gramicidine A (gA) at the same dimensional scale. The gA coordinates were taken from the literature [2] . Red ellipsoids (for TCT ) or balls (for gA) designate oxygen atoms, blue for nitrogen, grey for carbon and white for hydrogen. Full size image X-ray structure of TCT The crystal structure reveals that the intertwined monomeric strands of TCT are held in double-helix form. The robustness of the double-helix results from the synergistic H-bonding between triazole moieties and hydrophobic interactions between the central –(CH 2 ) 6 – chains. This assembled pattern generates T- channels with an empty interior void averaging 5 Å in van der Waals diameter, very close to dimensional behaviours of the gA channel ( Fig. 1c ) [2] . The pore contains an inversion symmetry center with half-superior and half-inferior inner surfaces of opposite chirality. This results in the formation of aqueous-lubricated hour-glass channels of alternating tight ( d =2.5 Å) and large ( d =4 Å) free pore openings, considering the water molecule occupancy of ~1.2 Å. The water molecules are arranged into a helical array inside the T-channel and are mainly located in two positions to form –C=O···H w and –NH···O w H-bonds with the –C=O and –N-H groups pointing toward the centre of the channel, similar to that in gA [2] . Considering the electron density map of water molecules observed in crystal structure of TCT they can be really associated with a local water disorder/motion ( Supplementary Note 2 , Supplementary Fig. 3 ). These assumptions have been confirmed by thermal analyses ( Supplementary Fig. 4 ). Theoretical calculations To gain insight into the local structure of water, we performed Monte Carlo simulations. The axial density profile reveals significant ordering of confined water mostly located in two layers near to the surface of the T-channel ( Fig. 2a and Supplementary Fig. 5 ). The pair correlation functions between O W and H W exhibits short-range positional order, very close to liquid water. Moreover, these results show enhanced interactions between neighbouring water molecules than those interacting with inner groups at the surface of the T-channel ( Supplementary Fig. 6 ). The contour plots of the density of water molecules show two possible orientations of net dipole of water molecules within the T-channel and is mainly imposed by their strong interactions with the –C=O groups separated by the inversion centres pointing in the lower part towards + crystalographic axis, while in the upper part towards – crystalographic axis ( Fig. 2b and Supplementary Fig. 7 ). 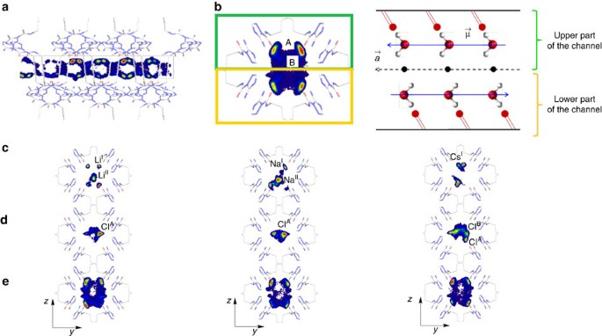Figure 2: Molecular simulations of water molecules and ions confined within T-channel. (a) Contour plots are showing the average density distribution of confined water molecules. The axial absolute density is readily obtained by multiplying the density corresponding to the probability of having a molecule in a slice with a volume unity, by the number of confined water molecules per T-channel. The density increases from blue, green, yellow, orange and red. The T-channel in stick representation has been added for clarity. (b) The radial density contour plot of water molecules located in two layers referring to position A (left and right side of the –C=O groups,R=1.0 Å) and position B (left and right side of the –N–H groups,R=2.1 Å). The orange and green boxes are the regions that are referred to as the lower and upper parts of the T-channel:μ>0 (that is, dipole pointing upward) andμ<0 (that is, dipole pointing downward) with respect to the crystallographic axis . The red double-bonded spheres correspond to the –C=O groups. The black dots represent the symmetry inversion centres while the dashed vector corresponds to the pore axis that is aligned with . The blue vectors illustrate the average net dipolar orientation of the water molecules, which are schematically shown to help in visualizing their average orientation. Contour plots showing the average density distribution of cations, (c) anions, (d) and of water molecules (e) in the presence of salts in the T-channel. Figure 2c,d show the contour plots of the average density for Li + , Na + , Cs + and Cl − ions, confined in the hydrated T-channel. For all cases, the Cl − density contours show pronounced axial maxima located near the –N–H groups. Li + , Na + and Cs + cations tend to be located close to the –C=O groups. The radial density contour plot for Li + exhibits a double layer structure (Li I and Li II ) with two maxima located in the centre ( R =1.75 Å) and close to the surface ( R =0.15 Å) of the T-channel. Similarly, Na + cations are located at 1.55 and 0.55 Å (Na I and Na II , respectively) due to the more important steric repulsion between the larger Na + cations. The larger Cs + occupies one position (Cs I located at 1.3 Å from the centre of the T-channel. The Cl A and Cl B identify the main locations occupied by the cations and the Cl − , respectively, in the T-channel [13] , [14] . The radial density contour plots show that Cl A layer is located at decreasing distances from the centre of the pore ( R =0.85, 0.65 and 0.5 Å for X =Li + , Na + and Cs + , respectively), which is due to steric repulsion as the cations become larger. Interestingly, in the case of CsCl, a second Cl B layer is observed in the centre of the T-channel. Figure 2: Molecular simulations of water molecules and ions confined within T-channel. ( a ) Contour plots are showing the average density distribution of confined water molecules. The axial absolute density is readily obtained by multiplying the density corresponding to the probability of having a molecule in a slice with a volume unity, by the number of confined water molecules per T-channel. The density increases from blue, green, yellow, orange and red. The T-channel in stick representation has been added for clarity. ( b ) The radial density contour plot of water molecules located in two layers referring to position A (left and right side of the –C=O groups, R =1.0 Å) and position B (left and right side of the –N–H groups, R =2.1 Å). The orange and green boxes are the regions that are referred to as the lower and upper parts of the T-channel: μ >0 (that is, dipole pointing upward) and μ <0 (that is, dipole pointing downward) with respect to the crystallographic axis . The red double-bonded spheres correspond to the –C=O groups. The black dots represent the symmetry inversion centres while the dashed vector corresponds to the pore axis that is aligned with . The blue vectors illustrate the average net dipolar orientation of the water molecules, which are schematically shown to help in visualizing their average orientation. Contour plots showing the average density distribution of cations, ( c ) anions, ( d ) and of water molecules ( e ) in the presence of salts in the T-channel. Full size image The pair correlation functions ( Supplementary Fig. 8 ) are consistent with three to ten times stronger interactions of the alkali cations and O W of water than those between the cations and –C=O groups. Despite such strong interactions, the alternative net-dipolar orientation of the confined water is preserved in the presence of all ion pairs with the average dipole orientation predominantly driven by the interaction with –C=O on the T-channel surface ( Supplementary Fig. 9 ). We anticipate that a dipolar water assisted ion-diffusion mechanism to be a starting point beside the known polarizable systems with electrostatic or steric asymmetry used until now to amplify ion diffusion [15] , [16] , [17] , [18] , [19] . Furthermore, it might provide useful information about the molecular-scale hydrodynamics of water [20] across the channels (see more details in Supplementary Notes 3 ). We performed experimental transport assays revealing that the T-channel presents water, proton and ion conduction, as well as cation/anion selectivity, properties similar to gA. The decrease in light scattering assessed by dynamic light scattering (DLS) [10] , [21] , is related to the increased water influx to vesicles in the presence of the T-channel ( Supplementary Fig. 10 ), with associated increase in mean vesicle radius ( Supplementary Fig. 11 ). The optical response is known to be very sensitive to the initial population of vesicles; a monodisperse vesicle preparation is required. Moreover, osmotic gradient and vesicle composition-related changes in vesicle shape make the scattering intensity a complex phenomenon [22] . Significant activity was observed within minutes of exposure to T-channels under osmotic stress conditions. Fifty times higher water transport activity ( k =6.0 × 10 −4 min −1 ) is obtained in the presence of T-channels compared with the control measurements where the dimethyl sulphoxide (DMSO) solvent was used ( k =1.3 × 10 −5 min −1 ). Control experiments showed that the T-channels operating without osmotic stress (NaCl loaded 1-palmitoyl-2-oleoyl-sn-glycero-3-phosphocholine (POPC) liposomes suspended in Na 2 SO 4 ) solution are inactive to the transport of water. The concentration of TCT added is well below the concentration that induces 5-(6-)carboxyfluorescein Na salt (CF) leakage under isotonic conditions (see Supplementary Figs 12 and 13 ), and we see no evidence of CF leakage in response to the osmotic gradients imposed in these experiments within the first few hours. The linear dependence of water transport rate as a function of TCT concentration ( Fig. 3a ) would be interpreted as progressive formation of robust transmembrane T-channels. The system is complex and response to the osmotic gradient could involve associated ionic fluxes to release entrapped electrolyte. In addition, the DLS experiment is complex and depends on the initial vesicle population distribution, lipid mixture and shape response to osmotic gradients [22] , [23] . Direct determination of changes in mean vesicle diameter by DLS similarly requires a monodisperse initial population. Swelling can be also observed in DOPC vesicles prepared using 0.1 M NaNO 3 in place of NaCl ( Supplementary Fig. 11 ). It is unlikely that this is physically reasonable as we do not know associated shape changes in this experiment. The size increases, but the magnitude of the change is not known. The complexities of the system require a fuller analysis of the population distribution and shape changes induced by the dual action of the TCT and the osmotic gradient. 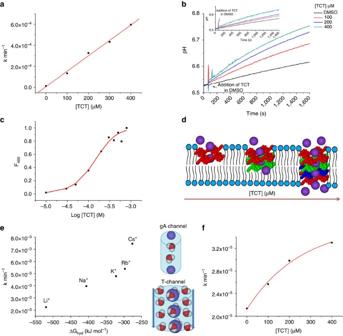Figure 3: Bilayer membrane transport experiments. (a) Water transport experiments. Linear rise of normalized rate constants,k, as a function of theTCTconcentration. (b) Proton transport experiments as determined in osmotic gradient assays and (inset) in non-osmotic gradient control assays. (c) Transport of Na+cations as determined in a pH gradient assay as a function of TCT concentration. (d) Possible hierarchical self-assembly of T-channels for increasingTCTconcentrations in the bilayer membrane. (e) The transport activity of T-channels versus dehydration energy of alkali cations show an increasing single-order exponential behaviour. The abrupt change in transport of low hydration energy cations (Cs+, Rb+), not observed for cation-water single file gA channels, involves double file dipolar water wires and ion wires along the T-channel. (f) Transport of Cl−anions as determined in a pH gradient assay. Non-linear rise of the Cl−transport rate constant values,k, as a function ofTCTconcentration. Figure 3: Bilayer membrane transport experiments. ( a ) Water transport experiments. Linear rise of normalized rate constants, k , as a function of the TCT concentration. ( b ) Proton transport experiments as determined in osmotic gradient assays and (inset) in non-osmotic gradient control assays. ( c ) Transport of Na + cations as determined in a pH gradient assay as a function of TCT concentration. ( d ) Possible hierarchical self-assembly of T-channels for increasing TCT concentrations in the bilayer membrane. ( e ) The transport activity of T-channels versus dehydration energy of alkali cations show an increasing single-order exponential behaviour. The abrupt change in transport of low hydration energy cations (Cs + , Rb + ), not observed for cation-water single file gA channels, involves double file dipolar water wires and ion wires along the T-channel. ( f ) Transport of Cl − anions as determined in a pH gradient assay. Non-linear rise of the Cl − transport rate constant values, k , as a function of TCT concentration. Full size image The change in internal pH under osmotic conditions ( Fig. 3b ) supports the assumption that the water T-channels in producing a water influx, also induce an efflux of protons towards the extravesicular solution ( Supplementary Fig. 14 ) [10] , [12] . The osmotic swelling causes vesicles to grow, thus altering the ionic balance between the lipids, which might be compensated by the absorption of ion pairs. Alternatively, proton-chloride symport could occur to directly increase the internal pH. Of the ion diffusion possibilities, proton mobility is expected to be the highest. The low proton transport activity observed under non-osmotic stress conditions strongly increases under osmotic gradient ( Fig. 3b , inset). It may occur according to the Grothuss mechanism [24] , along oriented water wires similar to that in gA channel [1] . This assumption is supported by the comparable O w –O W distances of 2.60 Å for an ideal Eigen cation [25] and of 2.75 Å observed in the crystal structure of TCT . Cation and anion transport through bilayer membranes was assessed by pH gradient assays [1] , [2] , [3] , [26] , [27] . The transport of Na + follows a typical does–response profile ( Fig. 3c and Supplementary Fig. 15 ) that gives an EC 50 of 140 μM for TCT compared with 1.2 pM for gA under comparable conditions. The Hill coefficients are very similar: 1.11±0.05 ( r 2 =0.993) for TCT and 1.02±0.10 ( r 2 =0.972) for gA ( Supplementary Figs 16–19 ). However, the fractional transport is a linear function concentration in the low concentration region for TCT with a positive intercept of (7.8±3.8) μM ( r 2 =0.991), while the comparable data for gA is non-linear in this region ( Supplementary Fig. 19 ). These are both so-called class II channels [17] . The gA result is consitent with prior literature, where rate-limiting insertion in vesicles has been proposed [18] . The TCT result indicates the formation of a stable pore that could be structurally characterized as we have done above ( Fig. 3d ) [17] . For the alkali cations, the transport activity increases in the order Li + <Na + <K + <Rb + <<Cs + , ( Fig. 3e and Supplementary Fig. 21 ) following the Eisenman sequence I corresponding to the energetic penalty for ion dehydration [28] . The net dipole moment of oriented water molecules inside the narrow gA pore influences the ionic conduction through a single-file of water cations, but dehydration energy seems to be more important as time, as the transport rates for Rb + and Cs + are the same [29] . In contrast, the cation-file permeation can be performed via successive hydration–dehydration processes along the parallel oriented water wires acting as an exceptional (bio)lubricant on the inner surface of the T-channel. The abrupt change in transport rate of low hydration energy cations (Cs + , Rb + ) is probably due to the more important contribution of dipolar ion diffusion along oriented water wires. The Cl − transport activity ( Fig. 3f and Supplementary Fig. 20 ) of k =3.2 × 10 −5 min −1 is two orders of magnitude lower than the transport activity of Na + of k =2.7 × 10 −3 min −1 . As with gA, which is totally impermeable to anions [3] , the dipolar distribution of charges and spatial disposition of water molecules at the interface with the inner backbone of the T-channel results in a significant increase of favourable hydration for cations, whereas they are not easily formed for anions. TCT concentrations about 1 mM support an exchange rate of 0.018 M min −1 comparable to other reported chloride transporters at this concentration [28] . Finally, the bilayer clamp technique [27] shows that the transport activity is slow to initiate, often requiring 40–60 min before the onset of activity ( Fig. 4 ). Once active conducting structures are formed, the activity continues to build in conductance over time, suggesting a progressive assembly of channels; late time activities can exceed 2 nS in conductance. Early periods of activity show 40% of open levels with transitions between them and the baseline, followed by quiescent periods and occasional bursts. Higher ( Fig. 4a ) or lower conductance levels ( Fig. 4b ) are observed, together with flickering states or some very long openings ( Fig. 4c ). The observed values lie below the conductance expected of an open water-filled pore of 2.5 Å diameter by a Hille analysis. The magnitude of the smallest observed openings (35 pS) are larger than those of gA channels (25 pS) under comparable conditions of lipid and electrolyte [31] , [32] . These regular activities are eventually subsumed in a rising level of activity ( Fig. 4d ). Once this behaviour becomes established, the system does not revert to the earlier on–off state. However, current histograms of sections of later data with conductance <350 pS show that specific levels are populated within the overall erratic envelope. We regard the late behaviour as simply the sum of many of the early behaviours as the aggregation process builds active structures within the membrane. Within these erratic multiple conductance states the system displays a K + /Cl − selectivity of 2.2 according to a Goldman–Hodgkins–Katz analysis [27] . The two open states are never an exact multiple of conductance of one another, suggesting that they are related by a relatively simple addition–subtraction of a component rather than multiple copies of a single species. Multiple conducting species are an example of the ‘supramolecular polymorphism’ [17] . From the perspective of a Hille analysis, the expected conductance of a channel of fixed radius decreases as the channel becomes longer [27] . We therefore equate the lower open conducting state with a fully assembled channel and the higher state with the same channel lacking one or more units. The differences between the snapshots of these species therefore relates to the exact conditions of bilayer thickness and fluidity, which would control, as in gA channels [33] , both the observed conductance via a length matching and the relative stability and dynamics of the interconversions via the self-assembly equilibrium. The bilayer conductance data is fully consistent with the T-channel model proposed, and bears close resemblance to gA single-channel conductance behaviour. 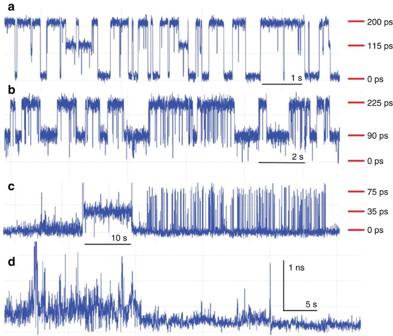Figure 4: Single channel conductance of T-channels under ‘early stage’ conductance records. (a)cis0.1 M/trans1 M KCl, diphytanoylphosphatidylcholine (diPhyPC), +120 mV; (b)cis0.1 M/trans1 M KCl, diPhyPC, +60 mV; (c) 1 M KCl, diPhyPC, +150 mV) and (d) ‘late-stage’ conductance record (1 M KCl, diphyPC, +100 mV). Figure 4: Single channel conductance of T-channels under ‘early stage’ conductance records. ( a ) cis 0.1 M/ trans 1 M KCl, diphytanoylphosphatidylcholine (diPhyPC), +120 mV; ( b ) cis 0.1 M/ trans 1 M KCl, diPhyPC, +60 mV; ( c ) 1 M KCl, diPhyPC, +150 mV) and ( d ) ‘late-stage’ conductance record (1 M KCl, diphyPC, +100 mV). Full size image In conclusion, T-channels provide a remarkable combination of functions very close to natural gA: water permeability, proton conductance via inner water wires, cation/anion selectivity and single-channel conductance. The single files of water acting as lubricant between the internal surface of T-channel and diffusing ions, imposes a net dipolar water orientation that influence the conduction of ions envisioned to diffuse along the dipolar hydrophilic wires. Such correlation between two simple dissymmetric properties, that is, the chiral inner pore superstructure [34] , [35] , [36] and oriented dipolar water wires, might contribute to conceive novel strategies for artificial ion diffusion processes. Conversely, the molecular-scale hydrodynamics of water and ionic species within such simple artificial channels could be of crucial relevance for other biological scenarios. Synthesis of compound TCT All reagents were obtained from commercial suppliers and used without further purification. 3-amino-1,2,4-triazole, 1 (5.75 g, 68.4 mmol) and 1,6-diisocyanatohexane, 2 (5 ml, 32.2 mmol) were dissolved in a mixture of 10 ml of THF, 5 ml of ethylacetate and 10 ml of N , N -dimethylacetamide, and refluxed at 120 °C for 15 min. Next, 50 ml of acetonitrile was added and the mixture was refluxed for 90 min and cooled to room temperature. Compound TCT , 3 (10.2 g, 30.4 mmol, 94%) precipitated as a pure white powder, was washed with methanol and dried. 1 H NMR (300 MHz, DMSO -d6 ): δ : 1.28 ( s , 2H); 1.51 ( t , 2H, 3 J =6.3); 3,17 (dt, 3 J =6.3 and 6.6, 2H); 7.17 ( s , 2H); 7.53 ( s , 1H); 8.21 ( t , 3 J =6.6, 1H) 13 C NMR (DMSO- d6 , 75 MHz): δ : 25.8; 28.9; 149.6; 150.9; 156.5. Mass spectrometry (electrospray ionization): m/z (%): 337.2 (100) [ TCT +H] + . Formation of liposomes Egg yolk L -α-phosphatidylcholine (EYPC chloroform solution, 600 μl, 790 μmol) or POPC chloroform solution (600 μl, 790 μmol) was dissolved in a CHCl 3 /MeOH mixture, the solution was evaporated under reduced pressure and the resulting thin film was dried under high vacuum for 2 h. The lipid film was hydrated in 1.2 ml of phosphate buffer (10 mM sodium phosphate, pH 6.4, 100 mM NaCl) containing 10 μM HPTS (pyranine, 8-hydroxypyrene-1,3,6-trisulphonic acid trisodium salt) for 40 min. During hydration, the suspension was submitted to at least five freeze–thaw cycles (liquid nitrogen, water at room temperature). The large multilamellar liposome suspension (1 ml) was submitted to high-pressure extrusion at room temperature (21 extrusions through a 0.1-μm polycarbonate membrane afforded a suspension of large unilamellar vesicles (LUVs) with an average diameter of 100 nm). The LUV suspension was separated from extravesicular dye by size-exclusion chromatography (stationary phase: Sephadex G-50, mobile phase: phosphate buffer) and diluted with the same phosphate buffer to give a stock solution with a lipid concentration of 11 mM (assuming 100% of lipid was incorporated into liposomes). Water transport experiments The water permeability were determined by using a DLS method and Zetasizer Nano Series S apparatus from Malvern. One hundred microlitres of vesicles stock solution, containing 10 mM of sodium phosphate buffer pH 6.4 and 100 mM of sodium chloride, are diluted in 1.9 ml of distilled water and stirred in a polystyrene cell. Twenty microlitres of DMSO stock solutions ( Supplementary Table 2 ) of 10–40 mM of TCT (final vesicle solution concentrations of 0.1–0.4 mM) are added causing water influx to vesicles. The decrease in light scattering (number of counts at 600 nm) is caused by vesicle swelling, which reduces the vesicle-medium contrast, and therefore the scattering was recorded at the following experimental conditions: t =25 °C, Position: 4.65 mm, Attenuator: 6, Dispersant: Water; R.I.: 1.33; Viscosity: 0.887, Record time: 60 s; Material R.I.: 1.59. Results were normalized to fit between zero and unity, and rate constants are calculated by using a linear fit model by subtracting the DMSO baseline observed in control experiments. Carboxyfluorescein leakage experiments EYPC chloroform solution (1 ml, 25 mg) was evaporated under reduced pressure and the resulting thin film was dried under high vacuum overnight. After hydration (>30 min) with 1 ml buffer (10 mM HEPES, 10 mM NaCl, 50 mM CF, pH 7.0), the resulting suspension was subjected to five freeze–thaw cycles (liquid N 2 ; 22 °C, water bath) and 15 times extruded through a polycarbonate membrane (pore size 100 nm). Extravesicular components were removed by size-exclusion chromatography (Sephadex G-50) with 10 mM HEPES, 100 mM NaCl, pH 7.0. Final conditions: ~2.5 mM EYPC; inside: 10 mM HEPES, 10 mM NaCl, 50 mM CF, pH 7.0; outside: 10 mM HEPES, 100 mM NaCl, pH 7.0. EYPC-LUVs-CF (25 μl, inside: 10 mM HEPES, 10 mM NaCl, 50 mM CF, pH 7.0) were added to 1,975 μl gently stirred, thermostated buffer (10 mM HEPES, 100 mM NaCl, pH 7.0) in a cuvette. The time-dependent changes in fluorescence intensity I t ( λ exc =492 nm, λ em =517 nm) were monitored for 240 seconds, with addition of TCT or gA at t =30 s, and addition of triton X-100 (50 μl 5% aq) at t =210 s. Time courses of I t were normalized to fractional intensities I f using the equation: I f =( I t − I 0 )/( I ∞ − I 0 ), where I 0 = I t at t =0 s and I ∞ = I t after lysis ( Supplementary Figs 11 and 12 ). Proton transport experiments One hundred microlitres of HPTS-loaded vesicles (stock solution) was suspended in 1.9 ml of milliQ water (osmotic gradient assay, Supplementary Fig. 14a ) or 1.9 ml sodium phosphate, pH 6.5 with 50 mM Na 2 SO 4 (non-osmotic gradient assay, Supplementary Fig. 14b ), and placed into a fluorimetric cell. The emission of HPTS at 510 nm was monitored with excitation wavelengths at 403 and 460 nm. During the experiment, 20 μl of a 0–40 mM DMSO solution of the compounds TCT was added at t =60 s. Maximal possible changes in dye emission were obtained at t =500 s by lysis of the liposomes with detergent (40 μl of 5% aqueous Triton X-100). The pH values were calculated for each point from the HPTS emission intensities according to the calibration equation pH 1.1684·log( I o / I 1 )+6.9807, where I o is the emission intensity with excitation at 460 nm and I 1 is emission intensity with excitation at 403 nm. At the end of experiment, the aqueous compartment of liposomes was equilibrated with extravesicular solution by lysis of liposomes with a detergent (40 μl of 5% Triton X-100). Cation transport experiments One hundred microlitres of HPTS-loaded vesicles (stock solution) was suspended in 1.9 ml of the corresponding buffer and placed into a fluorimetric cell. The emission of HPTS at 510 nm was monitored with excitation wavelengths at 403 and 460 nm simultaneously. During the experiment, 20 μl of a 0–40 mM DMSO ( Supplementary Table S2 ) stock solution of the compound TCT (final vesicle solution concentrations of 0.10, 0.20 and 0.40 mM) was added at t =0 s, followed by injection of 21 μl of 0.5 M aqueous NaOH at t =60 s. Addition of NaOH resulted in a pH increase of ~1 pH unit in the extravesicular buffer. Maximal possible changes in dye emission were obtained at t =500 s by lysis of the liposomes with detergent (40 μl of 5% aqueous Triton X-100). The experiment is ended at t =600 s. The final transport trace was obtained as a ratio of the emission intensities monitored at 460 and 403 nm, and normalized to 100% of transport. Pseudo-first-order rate constants were calculated from slopes of the plot of ln([H + ins ]−[H + out ]) versus time, where [H + ins ] and [H + out ] are the intravesicular and extravesicular proton concentrations, respectively. The [H + out ] was assumed to remain constant over the course of the experiment, while [H + ins ] values were calculated for each point from the HPTS emission intensities according to the calibration equation pH=1.1684·log( I o / I 1 )+6.9807, where I o is the emission intensity with excitation at 460 nm and I 1 is emission intensity with excitation at 403 nm. The absolute values for rate constants varied depending on the age of the vesicular solution and the actual stock solution of liposomes used. The ratios between absolute values of rate constants obtained from experiments on the same batch of liposomes, however, did not vary significantly. Anion transport experiments Fluorescence Method : One hundred microlitres of HPTS-loaded vesicles (stock solution) was suspended in 1.9 ml of an iso-osmotic phosphate sulphate buffer (10 mM sodium phosphate, pH 6.4, 75 mM Na 2 SO 4 ) and placed into a fluorimetric cell. The emission of HPTS at 510 nm was monitored with excitation wavelengths at 403 and 460 nm simultaneously. During the experiment, 20 μl of a 0–40 mM DMSO solution of the compound of TCT was added at t =60 s. Maximal possible changes in dye emission were obtained at t =500 s by lysis of the liposomes with detergent (40 μl of 5% aqueous Triton X-100). The pH values were calculated for each point from the HPTS emission intensities according to the calibration equation pH=1.1684·log( I 0 / I 1 )+6.9807, where I 0 is the emission intensity with excitation at 460 nm and I 1 is emission intensity with excitation at 403 nm. At the end of experiment, the aqueous compartment of liposomes was equilibrated with extravesicular solution by lysis of liposomes with detergent (40 μl of 5% aqueous Triton X-100). Electrochemical method : A chloroform solution of 8:1:1 PC:PA:cholesterol (Avanti Polar lipids) was dried under high vacuum pump. The internal buffer was prepared using 5.00 × 10 −4 M tris(hydroxymethyl) aminomethane, 0.1 M NaCl in deionized H 2 O, adjusted to pH 7.0 with HCl, made to 100 ml. The external buffer was prepared using 5.00 × 10 −4 M tris(hydroxymethyl)aminomethane, 0.1 M NaNO 3 in deionized H 2 O, adjusted to pH 7.0 with HNO 3 , made to 100 ml. The 50-mg dried lipid film was hydrated with 1 ml of the internal buffer. The solution was frozen using liquid nitrogen and allowed to thaw (repeated three times). The solution was then sonicated with an immersion probe (2 s pulses for 20 s, repeat three times) in a water and ice bath. The vesicles were then left overnight. The vesicles were then sized by extrusion (Avestin, polycarbonate membrane, pore diameter 400 nm, diameter 19 mm) with 19 passes. The buffer was then switched to the external nitrate buffer by size exclusion (PD-10 Sephadex G-25 column, GE Health Systems; rinsed with five volumes of external buffer). Once the first 3–4 cloudy drops had passed through the column, an ~1 ml fraction was collected. The ion selective electrode (ISE) system consisted of a glass-jacketed and -thermostated cell (25 °C) containing a double junction Ag/AgCl reference electrode with saturated KCl in the interior and the external buffer solution in the exterior compartments, and a solid-state chloride-specific electrode (Fisher Scientific). Potentials were monitored with a recording mV meter (Mettler automatic titrimeter driven by an Excel spreadsheet). The system was calibrated by preparing standards of known concentration (0.1 M, 0.01 M, 0.001 M, 0.0001 M, NaCl in H 2 O) using the external buffer. The standards were measured and a calibration curve was generated using activities calculated by an extended Debye–Huckel method [37] . To perform assays, external buffer (4 ml) in the cell was allowed to come to an equilibrium temperature before data collection was initiated. After 120 s, 150 μl of vesicle solution was injected into the vessel. At 240 s, the compound of interest was injected into the vessel. At 640 s, the vesicles were lysed using a surfactant (5% Triton X-100, deionized H 2 O). Data were collected until 760 s. The data saved in an Excel worksheet were converted from electrode potentials (mV) to activities using the calibration, and the first 200 s of activity–time data following compound injection was fit to a linear function to give a zeroth order rate constant ( Supplementary Table 3 ). The T-channel is also capable of supporting anion–anion exchange of chloride for nitrate. No quantitative comparison is possible with cation rates as the lipid mixture required differed from the experiments above; vesicles in these experiments used a ratio of 8:1 mixture of EYPC: egg phosphatidic acid:cholesterol and were prepared with 0.1 M entrapped NaCl, pH 7.0. Injection of this vesicle solution to 0.1 M NaNO 3 solution gave the steady release of chloride detected by a chloride-selective electrode. The channel under these conditions is equilibrated with water and sodium ions with both electrolytes buffered; hence, the process must involve chloride efflux accompanied by nitrate influx. Bilayer clamp experiment A model BC-535 A bilayer clamp (Warner Instrument Corp.) was used for all planar bilayer experiments. All data were hardware filtered at 1 kHz (8-pole Bessel filter), digitized (Axon 1440a) and recorded in a survey mode using the Gap-free protocol and processed (ClampEx and ClampFit 10.3.1.5). Chambers were made of Delrin holding a polystyrene cup with an aperture of 250 μm. The lipid was diphytanoylphosphatidylcholine (diPhyPC) (Avanti Polar lipids). A stock solution of 25 mg ml −1 lipid in CHCl 3 was dried under N 2 and then re-suspended in 100 μl decane. The electrolyte used was 1 M KCl, in 10 mM HEPES, 10 mM TRIS, pH 7 (unadjusted). The aperture was primed with 0.5–1 μl of decane/lipid and excess solvent was removed by blowing N 2 over the aperture. The cup was then placed into the electrolyte-filled holding cell, consisting of 5 ml and 3 ml chambers, and salt bridges (KCl/Agar) and electrodes (Ag/AgCl) were attached. Bilayers were formed by brushing on 1–1.5 μl of the decane/lipid mix over the aperture and were monitored for stability, capacitance and resistance for at least 20 minutes before test compound was added. Compound was added by injection from an organic solution (typically no more than 1–10 μl of solution) or by breaking the lipid-only bilayer and brushing on the compound preloaded in a lipid mix. Bilayers were tested repeatedly for capacitance and resistance. Once formed, ‘activity’ from pristine bilayers was never observed. For the cation/anion selectivity experiment, the cell was assembled with a gradient cis (0.1 M KCl) trans (1 M KCl; both sides buffered with 10 mM HEPES/10 mM TRIS). The episodic stimulation protocol of 29 sweeps of 5 s for the range −8.5 to 33.5 mV in 1.5 mV steps was sampled at 10 kHz. This experiment was done for the prolonged multiple opening activity ( Fig. 4d ), as this type of activity can persist for a very long time at a high frequency. Sweeps were averaged over 100 cycles, and a current voltage curve was generated using the mean current for each averaged sweep. A linear fit to this data gave the reversal potential as the intercept (+14.8 mV) from which the Goldman–Hodgkins–Katz equation gave the K + /Cl − selectivity of 2.2. Accession codes: The x-ray crystallographic coordinates for the TCT squeezed and the non-squeezed model structures deposited at the Cambridge Crystallographic Data Centre, under Accession codes CCDC 924256 and 924257, respectively. These data can be obtained free of charge from Cambridge Crystallographic Data Centre: ( http://www.ccdc.cam.ac.uk/data_request/cif ). How to cite this article: Barboiu, M. et al. An artificial primitive mimic of the Gramicidin-A channel. Nat. Commun. 5:4142 doi: 10.1038/ncomms5142 (2014).